Conformable amplified lead zirconate titanate sensors with enhanced piezoelectric response for cutaneous pressure monitoring The ability to measure subtle changes in arterial pressure using devices mounted on the skin can be valuable for monitoring vital signs in emergency care, detecting the early onset of cardiovascular disease and continuously assessing health status. Conventional technologies are well suited for use in traditional clinical settings, but cannot be easily adapted for sustained use during daily activities. Here we introduce a conformal device that avoids these limitations. Ultrathin inorganic piezoelectric and semiconductor materials on elastomer substrates enable amplified, low hysteresis measurements of pressure on the skin, with high levels of sensitivity (~0.005 Pa) and fast response times (~0.1 ms). Experimental and theoretical studies reveal enhanced piezoelectric responses in lead zirconate titanate that follow from integration on soft supports as well as engineering behaviours of the associated devices. Calibrated measurements of pressure variations of blood flow in near-surface arteries demonstrate capabilities for measuring radial artery augmentation index and pulse pressure velocity. Research over the last decade has established inorganic nanoparticles [1] , [2] , [3] , nanowires [4] , [5] , [6] and nanomembranes [7] as materials for high-quality electronic devices on unusual types of substrates, including plastic foils and rubber sheets [8] . A key opportunity and a realm ripe for further development and growth follows from an ability to integrate such technologies with the soft, curved contours of the human body [9] . Although semiconductor devices such as light-emitting diodes, solar cells and transistors have received much attention, application requirements often demand co-integration of other types of active materials and classes of components. Lead zirconate titanate (PbZr 0.52 Ti 0.48 O 3 , PZT), as one example, is a ferroelectric/piezoelectric material for ultrasonic transducers [10] , microelectromechanical devices and actuators [11] , as well as pressure [12] and strain [13] sensors, owing to its large piezoelectric and electromechanical coupling coefficients, high dielectric permittivity and significant remnant polarization [14] . Force sensing, mechanical energy harvesting and actuation represent promising possible roles in stretchable systems that interface with the body. Recent studies show the ability to build PZT-based piezoelectric systems for uses ranging from the measurement of deformations of neuronal cells [15] to harvesting of electrical power from motions of the heart, lung and diaphragm [16] . Alternative options include barium titanate [17] , zinc oxide [18] , [19] and other inorganics in nanostructured forms. An important, unexplored area for application of such materials is in the continuous monitoring of pressure transients associated with arterial blood flow. The traditional cuff sphygmomanometer is one of the oldest and most established diagnostic tools for blood pressure, but it is not well suited for continuous monitoring and yields only two basic pressure values: systolic (greatest heart contraction) and diastolic (greatest heart dilation) [20] . As a result, capabilities for use in observation during hypertensive treatment, in evaluation for hemodynamic effects of atherosclerotic risk factors or in projections of life-threatening cardiovascular events [21] are limited. A popular alternative, known as arterial tonometry, uses arrays of transducers that press against a radial artery to measure external blood pressure [22] . The transducers consist of dielectric capacitor structures formed in chip-scale geometries integrated with processing electronics. Pressure waves associated with blood flow appear as mechanically induced changes in capacitance. Enhanced embodiments exploit films of PZT in capacitor structures that connect to silicon metal oxide semiconductor field effect transistors (MOSFETs) for signal manipulation [23] . A drawback of such technologies for use on the skin follows from their planar, rigid formats. By consequence, monitoring schemes often require straps, tapes, pins or other mechanical fixtures that can cause irritation and discomfort during prolonged use. Another device architecture that provides improved mechanics and potential for measurement capabilities in this context uses polypropylene ferroelectret films bonded by epoxy to the gate electrodes of amorphous silicon thin-film transistors on flexible polyimide substrates [24] . This structure represents one of a variety of devices based on organic materials for the semiconducting [25] , [26] , [27] , [28] and/or piezoelectric [29] components. Others exploit conductive elastomers [30] , [31] , triboelectric effects [32] and air-gap capacitors [33] , with and without integrated organic transistors, to offer simple construction and natural compatibility with the skin. Systems that incorporate organic active materials, however, typically have slow response times, strongly temperature-dependent behaviours, uncertain fatigue and lifetime properties, sensitivity to parasitics and/or high operating voltages. Here we present inorganic materials, heterogeneous designs and theoretical models for an ultrathin, compact device capable of softly laminating on the skin with capabilities and modes of use that lie outside of the scope of the above-mentioned approaches. These systems are small (~1 cm 2 ), lightweight (2 mg), thin (25 μm) and capable of stretching (to ~30%, with system-level effective modulus of ~60 kPa) to conform to the skin, while providing high levels of pressure sensitivity (~0.005 Pa), fast response times (~0.1 ms), low hysteresis, superior operational stability and excellent fatigue properties. Ultrathin (400 nm) sheets of high-quality PZT serve as the active components of capacitor-type structures that connect to the gate electrodes of MOSFETs based on nanomembranes of silicon (SiNMs). Specifically, a SiNM n-channel MOSFET (that is, n-MOSFET) amplifies the piezoelectric voltage response of the PZT and converts it to a current output via capacitance coupling. Comprehensive electromechanical measurements and theoretical models provide complete descriptions of the principles of operation, including enhanced piezoelectric responses in PZT when mounted on soft substrates. Applications of the technology include skin-mounted sensors for measuring arterial pulse pressure waves and evaluating subtle motions of the throat associated with speech. Quantitative correlations of data from the former class of measurement to those of conventional devices suggest opportunities in continuous, non-invasive monitoring of pressure transients associated with arterial blood flow. Fabrication and design The sensor ( Fig. 1a ) consists of an array of square elements of PZT, collectively connected to the gate electrode of an adjacent SiNM n-MOSFET (inset; Fig. 1a ), all mounted on a thin elastomer substrate of silicone (Smooth-on, Ecoflex 0030, Platinum Cure Silicone Rubber), as further illustrated in Supplementary Fig. 1a . The n-MOSFET consists of heavily phosphorus-doped regions of the SiNM for source and drain, and a lightly boron-doped region for the channel. A cross-sectional view and simplified equivalent circuit appear in Fig. 1b,c , respectively. 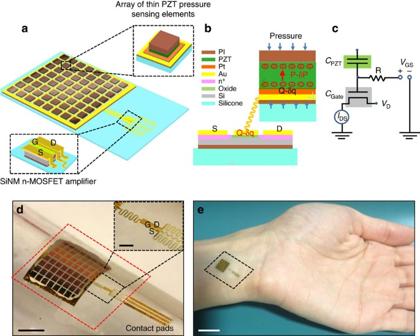Figure 1: Schematic illustrations and photographs of a thin conformable piezoelectric pressure sensor. (a) Illustration of the device, which includes a square array of piezoelectric thin-film transducers based on thin films of PZT (green; 400 nm), each encapsulated above and below with a layer of polyimide (PI) (brown; 3.6 μm for the top layer; 1.2 μm for the bottom layer) on square electrode pads of Pt (orange; 300 nm), interconnected by an underlying film of Au (gold; 150 nm), and supported by a silicone substrate (blue; 20 μm). The Au layer connects to the gate (gold; 150 nm) of a thin, field effect transistor by a stretchable, filamentary serpentine trace. The source (gold; 150 nm) and drain (gold; 150 nm) terminals of the transistor, which uses a silicon nanomembrane (grey) for the semiconductor, serve as the external output of the sensor. G, gate, S, source, D, drain of field effect transistor. (b) Cross-sectional schematic illustration of the pressure sensor and its connections to an associated transistor (also on a silicone substrate with 20 μm thickness). (c) Equivalent circuit for capacitance coupling between the pressure sensor and the transistor. (d) Photograph of a device wrapped on a cylindrical glass support. The red dashed box highlights the region that appears ina. Scale bar, 5 mm. The inset shows the serpentine traces and the transistor. Scale bar, 200 μm. (e) Photograph of a device laminated on a wrist. Scale bar, 2 cm. Figure 1d shows a photograph of a typical integrated device in which serpentine conducing traces (optical micrograph shown in inset, top right of Fig. 1d ) provide an ability to stretch the overall system. Anisotropic conductive film (ACF; Ellsworth Adhesives) serves as an interface to external power supplies and measurement systems, for application of voltage on the gate ( V GS ) and drain ( V DS ), and evaluation of current between drain and source ( I DS ). The conductive back side of the anisotropic conductive film cable is isolated with a thin layer of poly(dimethylsiloxane) (PDMS). A photograph of a device laminated on the wrist appears in Fig. 1e . Figure 1: Schematic illustrations and photographs of a thin conformable piezoelectric pressure sensor. ( a ) Illustration of the device, which includes a square array of piezoelectric thin-film transducers based on thin films of PZT (green; 400 nm), each encapsulated above and below with a layer of polyimide (PI) (brown; 3.6 μm for the top layer; 1.2 μm for the bottom layer) on square electrode pads of Pt (orange; 300 nm), interconnected by an underlying film of Au (gold; 150 nm), and supported by a silicone substrate (blue; 20 μm). The Au layer connects to the gate (gold; 150 nm) of a thin, field effect transistor by a stretchable, filamentary serpentine trace. The source (gold; 150 nm) and drain (gold; 150 nm) terminals of the transistor, which uses a silicon nanomembrane (grey) for the semiconductor, serve as the external output of the sensor. G, gate, S, source, D, drain of field effect transistor. ( b ) Cross-sectional schematic illustration of the pressure sensor and its connections to an associated transistor (also on a silicone substrate with 20 μm thickness). ( c ) Equivalent circuit for capacitance coupling between the pressure sensor and the transistor. ( d ) Photograph of a device wrapped on a cylindrical glass support. The red dashed box highlights the region that appears in a . Scale bar, 5 mm. The inset shows the serpentine traces and the transistor. Scale bar, 200 μm. ( e ) Photograph of a device laminated on a wrist. Scale bar, 2 cm. Full size image Device sensing properties Because the overall device involves coupled operation of two component parts, their separate characterization represents a natural starting point for analysis of the behaviours and underlying physics. Application of calibrated weights (post structures made of PDMS) to the PZT elements after coating their top surfaces with an electrode enables measurement of their responses to controlled pressures between 1 and 10 Pa, as in Supplementary Fig. 2 . 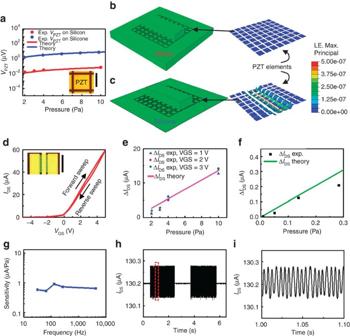Figure 2: Fundamental piezoelectric responses and performance data for the amplified pressure sensor. (a) Dependence ofVPZTon applied pressure for PZT sensors on a silicon wafer and on a soft silicone substrate. The inset shows a microscope image of a single PZT element in the array that makes up the sensor. Scale bar, 500 μm. The lines correspond to results from calculations based on analytical modelling and FEM. FEM results showing the modes of deformation of the PZT elements in the array, when mounted on (b) silicon and (c) silicone substrates with a scale factor of 106. LE, logarithmic strain. (d)IDSversusVGScharacteristics for a SiNM n-MOSFET with 200 μm channel width for forward and reverse bias sweeps (maximumIDShysteresis ~3 μA). The inset shows a microscope image of the device. Scale bar, 200 μm. Experimentally measured (symbols) and analytically calculated (lines) current response of an integrated sensor to sound pressure, when implemented using a SiNM n-MOSFET with (e) 200 μm channel width at various appliedVGSand (f) 800 μm channel width. (g) Response of a sensor with a SiNM n-MOSFET with 800 μm channel width as a function of sound frequency. (h)IDSmeasured using the sensor ingas a function of time during exposure to sound generated by a stereo speaker (turned on for 2 s and off for 1 s). (i) Data corresponding to the red dashed rectangular region inh. Exp., experimental. Figure 2a shows the voltages ( V PZT ) recorded for PZT devices built on a silicon wafer and on a silicone slab, both formed after transfer printing PZT films from their growth substrate. Multiple (50) measurements of the dependence of V PZT on applied pressure for a PZT sensor on silicone establish the high level of repeatability in the response ( Supplementary Fig. 3 ). It is immediately seen that the PZT devices on the silicone substrate offer responses that are more than two orders of magnitude greater than those of otherwise identical devices on silicon. Theoretical analysis yields a quantitative explanation. The dependence of the piezoelectric voltage on the contact force can be written ( Supplementary Note 1 ) Figure 2: Fundamental piezoelectric responses and performance data for the amplified pressure sensor. ( a ) Dependence of V PZT on applied pressure for PZT sensors on a silicon wafer and on a soft silicone substrate. The inset shows a microscope image of a single PZT element in the array that makes up the sensor. Scale bar, 500 μm. The lines correspond to results from calculations based on analytical modelling and FEM. FEM results showing the modes of deformation of the PZT elements in the array, when mounted on ( b ) silicon and ( c ) silicone substrates with a scale factor of 10 6 . LE, logarithmic strain. ( d ) I DS versus V GS characteristics for a SiNM n-MOSFET with 200 μm channel width for forward and reverse bias sweeps (maximum I DS hysteresis ~3 μA). The inset shows a microscope image of the device. Scale bar, 200 μm. Experimentally measured (symbols) and analytically calculated (lines) current response of an integrated sensor to sound pressure, when implemented using a SiNM n-MOSFET with ( e ) 200 μm channel width at various applied V GS and ( f ) 800 μm channel width. ( g ) Response of a sensor with a SiNM n-MOSFET with 800 μm channel width as a function of sound frequency. ( h ) I DS measured using the sensor in g as a function of time during exposure to sound generated by a stereo speaker (turned on for 2 s and off for 1 s). ( i ) Data corresponding to the red dashed rectangular region in h . Exp., experimental. Full size image where P is the contact pressure, A contact is the contact area between the PZT element and the weight, and α is a parameter that depends on the materials constants for PZT, as well as the deformation mechanics of each substrate. For the case of the wafer, deformation in the PZT involves approximately uniaxial compression along the thickness direction, as illustrated in Fig. 2b obtained using the Finite Element Method (FEM). This circumstance corresponds to , where t PZT is the thickness of PZT, A is the total area of PZT, including regions in direct contact with the weight and those not in contact, and e 33 , c 33 and k 33 are the piezoelectric, elastic and dielectric constants, respectively (see Supplementary Note 1 for details). FEM results confirm this relationship [34] ( Supplementary Fig. 4 ). For devices on silicone, the deformation in the PZT is complex and three-dimensional, as shown in Fig. 2c . Subsequently, the coefficient α is computed using FEM, giving a value of 0.068 V/N for the device layout ( Supplementary Fig. 5a,b ). For A =6 × 2 mm 2 as in experiments, Fig. 2a shows that equation (1) agrees well with measurements for both the silicon and silicone substrates, without any parameter fitting. This good agreement holds regardless of the contact location of the PDMS post on the array of PZT elements ( Supplementary Note 1 and Supplementary Fig. 5c–g ). The key finding is that the induced voltage associated with PZT on silicone is much larger than that on Si owing to the different modes of deformation. This is important as it yields approximately a 100-fold enhancement in sensitivity simply as a consequence of integrating devices of this type on compliant substrate, which is, in any case, required to allow soft lamination on the skin. We also note that the responses of the PZT elements associated with the pyroelectric effect ( Supplementary Fig. 6 ) are nearly two orders of magnitude smaller than the piezovoltages reported in Fig. 2a , for ranges of both temperature (25–35 °C) and pressure (4–10 Pa) that are relevant for cutaneous monitoring. As a result, effects of temperature can be ignored in the following. The piezoelectric voltage response from the PZT elements is further amplified by its integration with the flexible SiNM n-MOSFET. Figure 2d reveals I DS – V GS curves of representative transistors (channel width and length of 200 and 20 μm, respectively) that were measured in the common source configuration with a semiconductor parameter analyser (HP 4155C, Agilent) for values of V GS between 0 to 5 V in steps of 0.1 V at a V DS of 0.1 V. The full response corresponds to outputs measured at V DS from 0 to 5 V in steps of 0.1 V at different V GS ( Supplementary Fig. 7 ). Similar measurements on devices with channel widths of 200, 400, 600 and 800 μm appear in Supplementary Fig. 7 . Extracted electron mobilities lie in the range of 350–400 cm 2 V −1 s −1 and the on/off ratios exceed 10 5 . Unless otherwise noted, all of the results in the following use SiNM n-MOSFETs with 800 μm channel widths. The nature of the coupling between the PZT elements and the n-MOSFET can be understood by reference to the diagram in Fig. 1b and the simplified equivalent circuit in Fig. 1c . During use of the sensor, the n-MOSFET operates in an active mode, with V GS set to 3.5 V through a 100-MΩ resistor and V DS set to 0.1 V. This condition yields a transconductance ( g m ) of ~11 μA V −1 . Applying pressure to the PZT array generates a voltage owing to a decrease in the spontaneous polarization of PZT ( δP ) and a concomitant change in the compensating surface charge ( δq ), as indicated in Fig. 1b . Since the bottom electrode is shared with the gate of the n-MOSFET, redistribution of surface charge appears as a change in voltage on the gate (Δ V GS ), which is amplified by the action of the n-MOSFET. The equivalent circuit ( Fig. 1c ) involves a PZT capacitor in series with the gate oxide capacitor of the n-MOSFET. For such a series connection, modulation of the gate bias (Δ V GS ) with applied pressure is therefore related to V PZT as where C PZT and C Gox are the capacitances associated with the PZT and the gate oxide, respectively. For the devices examined here, C PZT / C Gox =0.15 × 10 6 (see Supplementary Note 2 for details). The change in current flow from drain to source is therefore Equations (1)–(3), ,  yield Δ I DS due to applied pressure as Δ I DS,pressure according to Measured values of Δ I DS,pressure under various applied pressures for a n-MOSFET with 200 μm channel width ( g m =11 μA V −1 ; Supplementary Note 3 ) appear in Fig. 2e . Equation (4) gives a linear relationship between Δ I DS,pressure and pressure, with a slope of Δ I DS,pressure / P =1.36 μA Pa −1 . Operation at various V GS (1, 2 and 3 V) yields consistent results, as a consequence of the nearly constant value of g m over this range ( Fig. 2d ). The device also exhibits low hysteresis behaviour, as seen in Supplementary Fig. 8a . Repeated application and release of pressure using the same setup ( Supplementary Fig. 2 ) show stable behaviour over 1,000 cycles ( Supplementary Fig. 8b ). Scaling studies of responses of separate sensors using SiNM n-MOSFETs with different channel widths (200, 400, 600 and 800 μm), and a fixed channel length (20 μm) indicate expected behaviours ( Supplementary Fig. 9 ). An audio speaker system (iHM79; Supplementary Fig. 10 ) enables examination of the sensor response under low pressures and high frequencies. Sound decibel levels (Radio Shack, 33–2055) recorded at the position (~1 cm from the speaker) of the sensor define the pressures ( Supplementary Note 4 ). Figure 2e shows a linear relationship between the sensor response and pressure, with a slope of ~2 μA Pa −1 . The I DS recorded during exposure to a middle C note (1 kHz, 80 dB) appears in Fig. 2f . The frequency response is the same over the audio range, as shown in Fig. 2g . The region highlighted by the red dashed box of Fig. 2h ( I DS measured using the sensor as a function of time during exposure of 1 kHz, 80 dB sound by a stereo speaker) is given in Fig 2i . The response time is ~0.1 ms ( Fig. 2i ), which exceeds requirements for pressure monitoring of blood vessels of the body. As illustrated in Supplementary Fig. 8c , the response remains the same under 1 kHz, 80 dB sound for 24 h. Mechanical stretchability and flexibility Serpentine traces for gate, drain and source and a silicone substrate allow stretching at the system level, without affecting the performance of the PZT arrays or the SiNM n-MOSFET. Supplementary Fig. 11 illustrates the ability of the device to accommodate 30% uniaxial strain, without any degradation in operating characteristics. Optical images and mechanics modelling of the serpentine traces illustrate reversible buckling during deformation, in a way that minimizes strains in the materials. For stretching up to 25%, the computed maximum principal strains in the Au are less than the failure strains (~5% for Au; ref. 35 ). At 30%, both experiment and simulation indicate fracture of certain parts of the serpentine ( Supplementary Fig. 11f ). Sensors with this construction can wrap easily around a finger or a pen, as in Fig. 3a,b , respectively. Bending-induced strains can, of course, influence the response of the sensor; such effects are important to understand, as they can influence the operation when mounted on the skin. Studies that involve mounting a sensor on cylindrical supports with different radii reveal the change in current flow from drain to source due to bending, Δ I DS,bending , as a function of tube radius ( Fig. 3c ). 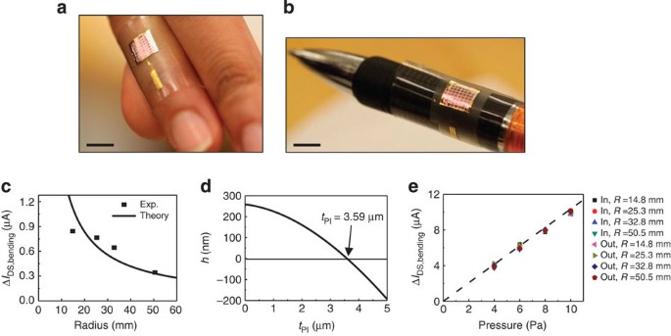Figure 3: Bending effect on a sensor that uses a SiNM n-MOSFET with 800 μm channel width. Photograph of a sensor wrapped on (a) a finger and (b) a pen. Scale bar, 1 cm. (c) Experimentally measured and theoretically calculated variations in ΔIDS,bendingwith bending radius for the sensor. (d) Distance from the NMP to the mid-plane of the PZT island (h) as a function of the thickness of top layer of PI (tPI). WhentPI=3.59 μm,h=0 mm and the effects of bending on the sensor response are minimal. (e) Variation in ΔIDS,pressureas a function of applied pressure for the sensor with different bending radii under different bending direction; Inward (In) and Outward (Out). Theory suggests that it is possible to write (see Supplementary Notes 5 and 6 for details) Figure 3: Bending effect on a sensor that uses a SiNM n-MOSFET with 800 μm channel width. Photograph of a sensor wrapped on ( a ) a finger and ( b ) a pen. Scale bar, 1 cm. ( c ) Experimentally measured and theoretically calculated variations in Δ I DS,bending with bending radius for the sensor. ( d ) Distance from the NMP to the mid-plane of the PZT island ( h ) as a function of the thickness of top layer of PI ( t PI ). When t PI =3.59 μm, h =0 mm and the effects of bending on the sensor response are minimal. ( e ) Variation in Δ I DS,pressure as a function of applied pressure for the sensor with different bending radii under different bending direction; Inward (In) and Outward (Out). Full size image where ē = e 31 −( c 13 / c 33 ) e 33 and are effective piezoelectric and dielectric constants, t PZT is the thickness of PZT element, R is the bend radius, h is the distance from the neutral mechanical plane (NMP) to the mid-plane of the PZT element ( Fig. 3d and Supplementary Fig. 12 ), where η depends on the bending stiffness ratio in the sections with and without the PZT elements and is given in the Supplementary Note 5 . The coefficient in equation (5) is for g m =33.2 μA Pa −1 and C Gox =3.72 pF; C PZT =0.14 μF; t PZT =400 nm; and h =1.19 nm, ē =−34 C m −2 , , and η =327 obtained from Supplementary Note 5 . As shown in Fig. 3c , equation (5) agrees reasonably well with experimental results, without any parameter fitting, and both show that Δ I DS,bendin g is inversely proportional to the bend radius R ( Fig. 3c ). Equation (5) implies a means to eliminate the effect of bending on pressure measurement from the Δ I DS,pressure – P relation in equation (4). In particular, with an appropriate value of t PI , h can be zero (that is, the NMP coincides with the mid-plane of the PZT layer), and therefore Δ I DS,bending =0. For the material properties and thicknesses used in experiments, a plot of h versus t PI ( Fig. 3d ) suggests that h =0 occurs when t PI =3.59 μm, which is close to the value used in experiments ( t PI =3.6 μm). For this t PI , Fig. 3e shows ΔI DS,pressure as a function of P for various outward (Out) and inward (In) bending radii. The data establish a linear relationship between Δ I DS,presssure and P with a coefficient of proportionality consistent with that in Fig. 2f . This behaviour is the same for all bend radii, ranging from 14.8 to 50.5 mm in Fig. 3c , that are larger than the in-plane dimensions of each PZT element (557 × 625 μm 2 , spacing of 170 μm). The conclusion is that the devices can measure pressure accurately on any body part with a radius of curvature larger than a few millimetres (for example the wrist). For sensors that do not use an NMP design, the relationship between ΔI DS,pressure and P remains linear, but with different coefficients of proportionality ( Supplementary Fig. 12b ). Blood pressure wave measurements and vibration detection Photographs of a sensor on the wrist appear in Fig. 4a,b . Demonstrations involved a healthy female in her late twenties, under approval by the Institutional Review Board of the University of Illinois (IRB no. 13561). No allergic reactions, redness or damage to the skin were observed in any of our studies. At a gate voltage of 3.5 V, without variation in pressure, the value of I DS is constant over time, as shown in Supplementary Fig. 13 . Changes in I DS result from variations in pressure associated with blood flow, as in Fig. 4c . The blood vessel examined here covers an area of ~0.6 × 0.2 cm 2 that affects ~20 PZT elements in the array. The region indicated by the dashed box of Fig. 4c appears in Fig. 4d . The peak labelled P 1 is the sum of the incident (ejected) wave and reflected wave (from the hand); P 2 is the peak of the reflected wave from the lower body minus end-diastolic pressure; P 2 / P 1 is the radial artery augmentation index (AI r ); and Δ T DVP is the time difference between these two peaks and represents a measure of arterial stiffness [36] . The measured values of AI r ~0.45 and Δ T DVP ~0.2 s are compatible with a person in their late twenties, as reported by Nichols via tonometry [37] . The device of Fig. 4a,b can also determine small variations in the diastolic tail of the pulse pressure wave; such features provide additional detailed information and are undetectable with conventional arterial tonometry [36] . The Δ I DS,pressure for P 1 corresponds ~4 Pa, with similar responses from sensors that use SiNM n-MOSFETs with different channel widths (400, 600 and 800 μm; Supplementary Fig. 14 ). As a further check of behaviour, poling the PZT in the opposite direction ( Supplementary Fig. 15 ) yields waveforms that have the same magnitudes but with forms inverted compared with those observed in Fig. 4c and Supplementary Fig. 14 . 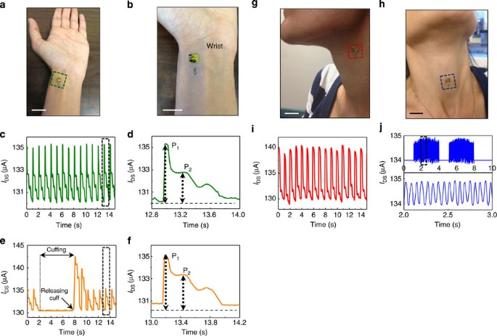Figure 4: Blood pressure wave measurements on the wrist and neck. Photograph of (a; scale bar, 2 cm) the sensor placed on a wrist for measuring fast transients in the pressure associated with flow of blood through near-surface arteries, (b; scale bar, 1 cm) magnified view. (c)IDS–time plot for a sensor mounted on the wrist. (d)IDS–time plot for data in the region indicated by the dashed box inc. (e)IDS–time plot for the sensor while reading pressure on the wrist before, during and after application of pressure on the arm using a commercial pneumatic cuff. (f)IDS–time plot for data in the region indicated by the dashed box ine. Photograph of a sensor placed on (g; scale bar, 1 cm) neck during measurement of transient blood pressure waves and (h; scale bar, 2 cm) the middle of the throat during speaking.IDS–time plot of the response of the sensor from (i) blood pressure from the neck and (j) vibrations of the throat (location in between croid cartilage and thyroid gland) associated with speech with recording of the subject’s overt responses (/a/) (top graph). The bottom graph corresponds to the black dashed rectangular region in top graph. Figure 4: Blood pressure wave measurements on the wrist and neck. Photograph of ( a ; scale bar, 2 cm) the sensor placed on a wrist for measuring fast transients in the pressure associated with flow of blood through near-surface arteries, ( b ; scale bar, 1 cm) magnified view. ( c ) I DS –time plot for a sensor mounted on the wrist. ( d ) I DS –time plot for data in the region indicated by the dashed box in c . ( e ) I DS –time plot for the sensor while reading pressure on the wrist before, during and after application of pressure on the arm using a commercial pneumatic cuff. ( f ) I DS –time plot for data in the region indicated by the dashed box in e . Photograph of a sensor placed on ( g ; scale bar, 1 cm) neck during measurement of transient blood pressure waves and ( h ; scale bar, 2 cm) the middle of the throat during speaking. I DS –time plot of the response of the sensor from ( i ) blood pressure from the neck and ( j ) vibrations of the throat (location in between croid cartilage and thyroid gland) associated with speech with recording of the subject’s overt responses (/a/) (top graph). The bottom graph corresponds to the black dashed rectangular region in top graph. Full size image The fast response time allows sensing of blood pressure during transient events, such as those associated with cuffing of the arm. The data of Fig. 4e correspond to measurements on the wrist between 0 and 2 s, cuffing the arm (Manual Inflate Blood Pressure Kit, Walgreens, model WC010) between 2 and 8 s and then releasing the cuff. The region indicated by the dashed box of Fig. 4e appears in Fig. 4f . P 2 / P 1 and Δ T DVP are ~0.45 and 0.2 s, respectively, consistent with Fig. 4d . Furthermore, the sensor can be placed on nearly any location on the body, including the neck ( Fig. 4g ) and throat ( Fig. 4h ), to allow measurement not only of blood pressure ( Fig. 4i ) but also vibrations associated with speech ( Fig. 4j ). The former shows that the peak shape of Fig. 4i is more rounded and the magnitude of P 1 is higher by ~75% than that in Fig. 4c due to carotid artery blood pressure [37] . Long-term pressure wave monitoring The complete pulse pressure waveform is known to provide valuable information for diagnostics and therapy of cardiovascular diseases such as arteriosclerosis, hypertension and left ventricular systolic dysfunction [37] , [38] , [39] , [40] . Many hemodynamic parameters such as arterial index, upstroke time, stroke volume variation and cardiac output can be directly calculated or estimated in real time from the pressure waveforms [41] , [42] . The type of skin-mounted sensor reported here provides a promising path towards long-term diagnostics based on this measurement. 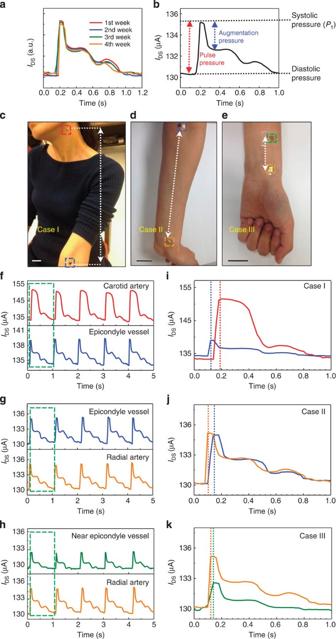Figure 5: Blood pressure wave monitoring over extended periods of time and determination of the PWV. (a) Normalized averageIDSresponse for ~15 single-pulse measurements collected once per week for a month (red: 1st, blue: 2nd, green: 3rd and orange: 4th week). (b) Average of the results inawith systolic, diastolic, pulse and augmentation pressure levels indicated. Photograph of two sensors placed on (c) the carotid artery of neck and lateral epicondyle vessel of the arm (Case I); (d) lateral epicondyle vessel and radial artery of the wrist (Case II); and (e) near epicondyle vessel and radial artery (Case III).IDS–time plot for (f) Case I, (g) Case II and (h) Case III, respectively. Scale bar, 3 cm. (i–k)IDS–time plot of data corresponding to the green dashed rectangular region inf–h, respectively. The time shifts of the initial peaks in the waveforms are indicated with dashed lines. Figure 5a shows measured waveforms, normalized to the first measured response, for weekly measurements over the course of a month. Corresponding blood monitoring results (an average systolic pressure of 110 mm Hg and diastolic pressure of 65 mm Hg; Blood Pressure Dock BP3, iHealth Lab Inc.) are shown in Supplementary Fig. 16 . Systolic, diastolic and pulse pressure conversion factors are ~0.81, ~0.50 and ~9 mm Hg μA −1 , as shown in Fig. 5b . These conversion factors correspond to the observed I DS values as systolic (~135 μA), diastolic (~130.5 μA) and pulse pressure (~4.5 μA). The collective results in Supplementary Fig. 17 suggest that the sensor is robust and suitable for long-term monitoring. Data on three human subjects (each in their early twenties) were collected with a 2-min interval in between four consecutive measurements, while the subjects were in a relaxed state and the blood pressure remained relatively constant. A analysis summary appears in Supplementary Fig. 17d,e . Supplementary Figure 18a–c shows measured waveforms, normalized to the first measured response, for weekly measurements on these three subjects. The repeatability in the pulse wave velocity (PWV) and the AI r ( P 2 / P 1 :(AI r )) is consistent with insignificant variations in blood pressure over this same period (measured with a cuff device). Simultaneous use of multiple sensors at different locations enables determination of the PWV. PWV is accepted as the most simple, robust and reproducible method to determine the regional arterial stiffness [43] . PWV is important because it can be quantitatively related to BP when calibrated using a conventional blood pressure cuff measurement device [44] . Calculating the PWV involves measurements at two sites with a known distance between them. This distance divided by the time separation associated with a given feature (for example, P 1 ) in the waveform defines the PWV. Figure 5c–e presents pictures of three cases: Case I: sensors on the carotid artery and the lateral epicondyle vessel; Case II: on the lateral epicondyle vessel and the radial artery of the wrist; and Case III: on the near epicondyle vessel and the radial artery of the wrist; respectively. PWV profiles of Cases I, II and III appear in Fig. 5f–h . As seen in Fig. 5i–k , PWV Case I is ~5.4 ms −1 where the distance between sensors is ~43 cm and time difference is ~0.08 s; PWV Case II is ~5.8 ms −1 where the distance between sensors is ~23 cm and time difference is ~0.04 s; and PWV Case III is ~6.5 ms −1 where the distance between sensors is ~6.5 cm and time difference is ~0.01 s. These PWV values are comparable with the typical aortic PWV (~4.5 ms −1 ) measured by tonometry in a healthy 20-year-old person [45] . Figure 5: Blood pressure wave monitoring over extended periods of time and determination of the PWV. ( a ) Normalized average I DS response for ~15 single-pulse measurements collected once per week for a month (red: 1st, blue: 2nd, green: 3rd and orange: 4th week). ( b ) Average of the results in a with systolic, diastolic, pulse and augmentation pressure levels indicated. Photograph of two sensors placed on ( c ) the carotid artery of neck and lateral epicondyle vessel of the arm (Case I); ( d ) lateral epicondyle vessel and radial artery of the wrist (Case II); and ( e ) near epicondyle vessel and radial artery (Case III). I DS –time plot for ( f ) Case I, ( g ) Case II and ( h ) Case III, respectively. Scale bar, 3 cm. ( i – k ) I DS –time plot of data corresponding to the green dashed rectangular region in f – h , respectively. The time shifts of the initial peaks in the waveforms are indicated with dashed lines. Full size image Results presented here demonstrate the ability to exploit enhanced piezoelectric effects in PZT elements on soft supports for precision, skin-mounted sensors for pressure. When coupled to SiNM-based field effect transistors, these devices offer unique capabilities in accurate measurements of subtle effects of motion on the surface of the skin, ranging from blood pressure pulse waves in near-surface arteries to vibrations on the throat associated with speech. The thin, conformal nature of the devices, together with their predictable responses, consistent with theoretical models, offer high performance operation, without measurable side effects during use in daily activities. The collective results suggest that these materials and the resulting sensor capabilities could be valuable for a range of applications in continuous health/wellness monitoring and clinical medicine. Current work focuses on long-term device characterization and wireless communication. Fabrication of SiNM MOSFETs The fabrication began with a silicon-on-insulator (top silicon thickness ~300 nm, p-type, SOITEC, France) wafer, consisting of lightly p-type doped (1 × 10 15 per cm 3 ) top silicon and a 1-μm-thick buried silicon dioxide (SiO 2 ) layer, as shown in Supplementary Fig. 1a . Cleaning the silicon-on-insulator wafers involved removal of organic and ionic contaminants by sequential immersion in: (1) 1:1:5 solution of NH 4 OH (ammonium hydroxide):H 2 O 2 (hydrogen peroxide):H 2 O (de-ionized (DI) water) at 80 °C for 10 min; (2) 1:50 solution of HF (hydrofluoric acid, 49%):(DI water) for 1 min; and (3) 1:1:6 solution of HCl (hydrochloric acid):H 2 O 2 :H 2 O (DI water) at 80 °C for 10 min. Thermal oxidation produced a layer of SiO 2 on the top silicon, as a mask for phosphorous doping. This thermal oxide was patterned by reactive ion etching (RIE; Plasma-Therm) with CF 4 /O 2 through a photoresist (PR) mask. The wafer was then cleaned with acetone and isopropyl alcohol to remove the remaining PR. Another RCA cleaning preceded solid state diffusion doping of phosphorous (2 × 10 20 per cm 3 ) in a 6-inch tube furnace (Lindberg/Tempress Model 8500 Dual-Stack Diffusion/Oxidation Furnaces) at 1,000 °C. A series of wet-etching steps using HF (49%) and piranha solution (3:1=H 2 SO 4 (sulphuric acid):H 2 O (DI water)) eliminated surface contamination. The top silicon was then patterned by RIE to form an array of 3 μm diameter circular openings. Immersion in HF (49%) removed the buried oxide to allow transfer printing of the resulting SiNM via a PDMS stamp onto a carrier wafer with a spin-cast layer of polyimide as an adhesive and an underlying layer of poly(methylmethacrylate) (495 A2). The SiNM was then patterned by RIE to define active regions for transistors. The gate dielectric consisted of a sandwich structure of SiO 2 (140 nm thick) with aluminium oxide (Al 2 O 3 ; 10 nm thick) above and below; the Al 2 O 3 is in contact with the Si. The SiO 2 and Al 2 O 3 were deposited by plasma-enhanced chemical vapour deposition (Plasma-Therm/Unaxis SLR730) and by atomic-layer deposition (Cambridge Nanotech), respectively. The gate dielectric was patterned by etching in buffered oxide etchant (BOE) (6:1). Deposition of 5 nm of Cr and 150 nm of Au followed by wet etching of the Au (Transene Company Inc., USA) and the Cr (OM Group, USA) defined electrodes aligned to the silicon and gate dielectric. The entire device was then encapsulated with a 1.2-μm-thick layer of PI to position the SiNM near the NMP. Etching the underlying PI with an O 2 plasma (Asher (LFE)) exposed the poly(methylmethacrylate) layer to enable its removal in hot acetone (110 °C) and to partially release the device, with PI above and below, from the wafer. The entire structure was then retrieved onto a piece of PDMS and pressed against a 20-μm-thick silicone (Smooth-on, Ecoflex 0030, Platinum Cure Silicone Rubber) substrate. A bilayer of 4 nm of Ti and 40 nm of SiO 2 deposited onto the back side of the device while on the PDMS enabled formation of strong bonds to the silicone. As a final step, the device, with bonded silicone, was transfer printed to a 200-μm-thick layer of poly(vinylalcohol) (A-30031, Best Triumph Industrial Ltd). Integration onto the skin involved placing the sensor on a transparent plastic frame and physically laminating the sensor on the skin. Rinsing with water removed the poly(vinylalcohol), leaving an ultrathin device in intimate, conformal contact with the skin. Devices mounted in this way exhibited excellent compliance and ability to follow skin motion without constraint or delamination. The plastic frame facilitated removal and re-application for repeated measurements. Separate adhesives were not needed to bond the devices to the skin. The adhesion strength was measured using a digital force metre (Mark-10, USA), using the following procedures [46] : the wrist was secured and the device substrate was connected to a force metre. The device was peeled away at a maximum speed of 1,000 mm min −1 in an upward direction, parallel to the width of the device, at room temperature. The maximum value of the force during this process defined the adhesion force. A typical device with a 20-μm-thick silicone substrate and lateral dimensions of ~1.5 cm (length) × 1 cm (width) showed an average adhesion force of 0.032 N. Photographs collected during mounting and peeling appear in Supplementary Fig. 19 . Fabrication of arrays of PZT capacitor structures The PZT was formed by sol–gel techniques on an oxidized silicon wafer coated with Pt/Ti (300 nm/20 nm). The PZT (INOSTEK; thickness 400 nm) was formed by a sol–gel process on an oxidized silicon wafer coated with Pt/Ti (300 nm/20 nm), following the procedures of Li et al . [47] A 0.4-M precursor solution consisted of zirconium n-propoxide, titanium isopropoxide and lead acetate trihydrate with acetic acid and propyl alcohol as the solvents. The prepared solution was spin-cast onto the Pt/Ti/SiO2/Si (100) substrate at 3,000 r.p.m. for 40 s. Pyrolysis and pre-crystallization occurred at 400 °C for 20 min. After deposition of five consecutive layers in this fashion, the sample was annealed at 680 °C for 10 min. The total thickness of the PZT was ~400 nm. The array of PZT elements consisted of square regions 557 × 625 μm 2 with a spacing of 170 μm formed by wet chemical etching in HNO 3 :BHF:H 2 O (nitric acid: buffered HF:DI water=4.51:4.55:90.95 through a hard-baked mask of PR (AZ4620, Clariant) as shown in Supplementary Figs 1b and 20 . The spacing facilitates access of concentrated HF for undercut etching of the PZT elements. The array structure provides a large sensing area. The hard baking process involved 80 °C for 5 min, 110 °C for 30 min and 80 °C for 5 min. The bottom Pt/Ti electrode was patterned by etching in HCl:HNO 3 :H 2 O(DI water)=3:1:4 at 95 °C also through a hard-baked mask of AZ4620. A layer of PI was spin cast on the sample at a thickness (3.6 μm) to position the PZT at the NMP. The PI was removed by O 2 plasma (Asher (LFE)) everywhere except for regions with sizes of 650 × 550 μm 2 centred on the PZT. These structures were protected by a PR mask during partial removal of the underlying SiO 2 with diluted HF (H 2 O:HF (49%)=1:3). The hard-baked PR was then removed in acetone (3 h). The fabrication yield was ~80%, limited mainly by cracking that sometimes occurred during the retrieval stage of transfer printing the PZT. Transfer printing PZT structures on a stretchable substrate As illustrated in Supplementary Fig. 1b , a PDMS stamp retrieved the partially undercut PZT/PI/Pt structures and delivered them to a layer of silver epoxy (Ted Pella Fast Drying Silver Paint (160040-30)) coated on an extended gate electrode of a SiNM n-MOSFET. The PZT elements bond at their base regions to a uniform conductive coating Ted Pella Fast Drying Silver Paint (160040-30) applied to an extended gate electrode of a SiNM n-MOSFET. This arrangement electrically connects the bottom Pt electrodes of the PZT elements. A 3.6-μm-thick layer of PI applied to the entire array locates the NMP at the mid-plane of the PZT ( Fig. 1a,b ). The choice of thickness involved balanced considerations in bendability, where thinner is better, and in voltage output, where thicker is better. A thickness of 400 nm represents a good choice. Investigation of properties of PZT and the device responses PZT capacitor structures with Ti/Pt (20 nm/300 nm) bottom electrodes and Cr/Pt (10 nm/200 nm) top electrodes were poled at 100 kV cm −1 for 2 h at 150 °C. Afterward, the top electrode was removed by etching the chromium and platinum. X-ray diffraction (Philips X'pert) was used to confirm the crystal structure of PZT, corresponding to two main peaks, belonging to (100) and (111) as seen in Supplementary Fig. 21a . A scanning electron microscope (Hitachi S4800) was used to examine cross-sections of the device stacks on a silicon wafer with the SiO 2 sacrificial layer and the underlying silicon substrate, as in Supplementary Fig. 21b . The hysteresis loop of the PZT in Supplementary Fig. 21c was obtained by using a ferroelectric tester (Radiant Technologies, Inc.). A semiconductor parameter analyser (4155C, Agilent) was used to characterize the SiNM n-MOSFETs and to perform open-loop voltage measurements for the response of the pressure sensor. The signal-to-noise ratios for typical measurements are ~50 ( Supplementary Fig. 22 ). PDMS posts served as calibrated weights in the milligram range, for applying well-defined levels of pressures to the PZT elements. A computed map of contact pressure between a representative post (1 mm thick) and an array of PZT elements on silicone appears in Supplementary Fig. 23 . Each PDMS post was placed on the PZT region with a vacuum tweezers with bent metal probe, 1-inch long, 3/32-inch cup diameter (Ted Pella, Inc., Vacuum Pickup System, 115 V) from a fixed distance. The voltage response to changes in temperature was investigated using the continuous heating method, with a heating rate of 1 °C min −1 . A small stage (All Electronics Corp.; 40 × 44 mm 2 ) was used to measure effects of temperature on the PZT active region of a device. Human subject demonstrations were performed under approval by the Institutional Review Board of the University of Illinois (IRB no. 13561). The informed consent was obtained from all subjects in human trials. How to cite this article: Dagdeviren, C. et al . Conformable-amplified lead zirconate titanate sensors with enhanced piezoelectric response for cutaneous pressure monitoring. Nat. Commun. 5:4496 doi: 10.1038/ncomms5496 (2014).